Farnesoid X receptor inhibits glucagon-like peptide-1 production by enteroendocrine L cells Bile acids are signalling molecules, which activate the transmembrane receptor TGR5 and the nuclear receptor FXR. BA sequestrants (BAS) complex bile acids in the intestinal lumen and decrease intestinal FXR activity. The BAS–BA complex also induces glucagon-like peptide-1 (GLP-1) production by L cells which potentiates β-cell glucose-induced insulin secretion. Whether FXR is expressed in L cells and controls GLP-1 production is unknown. Here, we show that FXR activation in L cells decreases proglucagon expression by interfering with the glucose-responsive factor Carbohydrate-Responsive Element Binding Protein (ChREBP) and GLP-1 secretion by inhibiting glycolysis. In vivo , FXR deficiency increases GLP-1 gene expression and secretion in response to glucose hence improving glucose metabolism. Moreover, treatment of ob/ob mice with the BAS colesevelam increases intestinal proglucagon gene expression and improves glycaemia in a FXR-dependent manner. These findings identify the FXR/GLP-1 pathway as a new mechanism of BA control of glucose metabolism and a pharmacological target for type 2 diabetes. Bile acids (BAs) are amphipathic molecules derived from cholesterol, synthesized and conjugated in the liver, stored in the gallbladder, expelled in the intestinal lumen after meal ingestion and further metabolized by the gut microbiota into secondary BAs. Initially considered to be dietary lipid detergents, BAs are now recognized as signalling molecules which, through binding and activation of the membrane receptor TGR5, the nuclear receptors vitamin D receptor, Pregnane X Receptor and Farnesoid X Receptor (FXR, NR1H4 ), play key roles in the control of energy homeostasis [1] . Secondary bile acids are more potent ligands for TGR5 (affinity for TGR5: LCA>DCA>CDCA>CA) than for FXR (affinity for FXR: CDCA>DCA=LCA>CA) (for review, see refs 1 , 2 ). TGR5, a G protein-coupled receptor, first described as a regulator of cytokine production in a human monocyte cell line [3] , was also shown to promote glucagon-like peptide-1 (GLP-1) secretion in response to BA by intestinal enteroendocrine L cells [4] . Although representing <1% of the intestinal epithelial cells, enteroendocrine cells play key roles in the regulation of energy metabolism through their capacity to secrete various bio-active peptides. After food ingestion, the incretins GLP-1 and glucose-dependent insulinotropic polypeptide are secreted by L and K cells, respectively, and subsequently potentiate postprandial insulin secretion by pancreatic β cells in response to glucose, the so-called incretin effect [5] . Even though the insulinotropic property of GLP-1 is maintained, its secretion in response to a meal is decreased in type 2 diabetic patients [6] , [7] . This observation has led to the development of DPP-IV inhibitors that increase GLP-1 half-life and GLP-1 mimetics, which improve glucose homeostasis with less risk for hypoglycemia. Together with TGR5, FXR controls BA-induced signalling pathways. FXR, predominantly expressed in the liver and intestine, was first identified as a regulator of hepatic BA metabolism through the induction of small heterodimer partner (SHP) in the liver and fibroblast growth factor 15 (FGF15) in the intestine, resulting in the subsequent inhibition of the rate-limiting enzyme in hepatic BA synthesis, cholesterol 7α-hydroxylase (CYP7A1) and the regulation of BA transporters (for review, see refs 8 , 9 ). FXR in the liver also plays a modulatory role in the regulation of lipid and glucose homeostasis. FXR activation with the synthetic agonist GW4064 decreases hepatic gluconeogenic gene expression and increases glycogenesis [10] thus improving glucose homeostasis in diabetic mice. In the postprandial state, FXR activation in hepatocytes also inhibits the induction of glycolytic gene expression by glucose through negative interference with the carbohydrate response element binding protein ChREBP (also known as MlxIPL) [11] , [12] . Recent studies have highlighted a metabolic role of non-hepatic and specifically intestinal FXR in mice under pathophysiological conditions such as obesity [13] , [14] , [15] , [16] . Indeed, oral treatment of high-fat-diet-fed mice with GW4064 promotes hyperglycaemia and obesity [13] , whereas an opposite effect is observed upon intraperitoneal injection of the drug [10] . Moreover, in two different models of obesity, whole-body FXR deficiency improved metabolic parameters, an effect not observed in hepatocyte-specific FXR-deficient animals [14] . Furthermore, intestinal specific FXR-deficient mice are protected against diet-induced obesity and non-alcoholic fatty liver disease [15] , [16] . These studies also identified a crucial role of the intestinal microbiota in BA signalling by regulating the ratio of BAs with agonist or antagonist activity on FXR. Indeed, the primary BA tauro beta-muricholic acid (TβMCA), whose levels are elevated in germ-free (GF) mice, acts as an FXR antagonist to improve glucose metabolism via intestinal FXR [15] , [17] . Finally, BA pool composition is modulated by BA sequestrants (BAS) (for review, see ref. 18 ). BAS, such as colesevelam, are anion exchange resins that trap BAs in the intestinal lumen. Initially used for their cholesterol-lowering effects, they have more recently been shown to act as antidiabetic drugs [2] , [14] , [19] . In diabetic db/db mice, BAS administration deactivates intestinal FXR and increases glucose clearance in peripheral tissues [19] . Among the proposed action mechanism of BAS is a TGR5-mediated increase of GLP-1 secretion in diet-induced obese mice [20] , [21] . In addition to their acute effects on GLP-1 secretion, BAS-bound BAs enhance proglucagon gene expression through TGR5, another mechanism via which this transmembrane receptor regulates GLP-1 production [20] . Whether FXR is expressed and plays a role in L cells has not been reported yet. Using the murine GLUTag L cell line, human intestinal biopsies and different mouse models, we demonstrate that FXR is expressed and functional in enteroendocrine L cells. In mice and in human ex vivo intestinal biopsies, activated FXR downregulates proglucagon mRNA levels. In vitro , FXR activation decreases both proglucagon mRNA and protein levels by interfering with ChREBP-mediated glucose-induction of proglucagon mRNA levels. FXR activation also inhibits the glycolysis pathway translating into decreased intracellular ATP levels, contributing to a decreased GLP-1 secretion in response to glucose. In vivo , FXR deficiency increases proglucagon mRNA levels and glucose-induced GLP-1 secretion in chow diet-fed mice, whereas the protective effect of FXR deficiency on glycaemic control in high-fat-fed mice is blunted by the GLP-1 receptor (GLP-1R) antagonist Exendin-4(9-39). Finally, treatment of ob/ob mice with colesevelam improves glycaemia at least in part by an FXR-dependent increase of proglucagon mRNA levels. FXR decreases proglucagon mRNA levels in mice and humans Previous studies have reported high expression of FXR in intestinal epithelial cells [22] , [23] . However, its expression in enteroendocrine L cells has not yet been assessed. We analyse Fxr expression in L cells sorted by fluorescence-activated cell sorting (FACS) from transgenic proglucagon-VENUS mice [24] , [25] . FACS-sorted L+ cells were separated from L cells with a purity >95% (ref. 24 ). As expected, the Fxr gene is more abundantly expressed in ileal non-L cells (ileum L−) than in colonic non-L cells (colon L−) ( Fig. 1a ). Surprisingly, compared with non-L cells, Fxr expression is higher in L cells from the ileum (ileum L+) and, albeit nonsignificantly, the colon (colon L+) ( Fig. 1a ). Confocal microscopy analysis on human intestinal biopsies reveal that FXR is expressed in GLP-1-positive cells from the jejunum ( Fig. 1b , Supplementary Movie 1 ) and colon ( Supplementary Fig. 1a ). 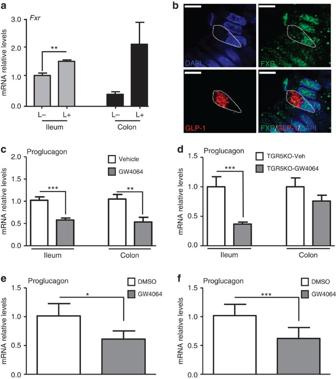Figure 1: FXR decreases proglucagon mRNA levels in mice and in human. (a)Fxrexpression by qPCR in FACS-sorted proglucagon-negative and proglucagon-positive cells from the ileum (ileum L−; ileum L+) and colon (colon L−; colon L+) of GLU-VENUS mice (n=3). (b) Twelve-micrometre-thick slices from human jejunal biopsies were incubated with antibodies against FXR (in green) and GLP-1 (in red). Nuclei are in blue. Co-expression in GLP-1-positive cells (dotted line) was assessed on a confocal microscope. Representative of three different FXR/GLP-1 immunostaining experiments. Scale bar, 2 μm. Proglucagon qPCR on cDNA from ileum and colon of 8-week-old wild-type (c) or Tgr5−/−(d) mice treated by gavage for 5 days with GW4064 (30 mpk;n=5 mice per group. Data are represented as mean ±s.d. (e) Proglucagon qPCR on cDNA from isolated primary intestinal epithelial cells from two wild-type miceex vivotreated for 24 h with DMSO or with GW4064 (5 μmol l−1). (f) Proglucagon qPCR on cDNA of human jejunal biopsies from four normoglycemic patientsex vivotreated for 16 h with DMSO or with GW4064 (5 μmol l−1). Data are represented as mean ±−s.e.m. Student’st-test, *P≤0.05, **P≤0.01 and ***P≤0.001. Figure 1: FXR decreases proglucagon mRNA levels in mice and in human. ( a ) Fxr expression by qPCR in FACS-sorted proglucagon-negative and proglucagon-positive cells from the ileum (ileum L−; ileum L+) and colon (colon L−; colon L+) of GLU-VENUS mice ( n =3). ( b ) Twelve-micrometre-thick slices from human jejunal biopsies were incubated with antibodies against FXR (in green) and GLP-1 (in red). Nuclei are in blue. Co-expression in GLP-1-positive cells (dotted line) was assessed on a confocal microscope. Representative of three different FXR/GLP-1 immunostaining experiments. Scale bar, 2 μm. Proglucagon qPCR on cDNA from ileum and colon of 8-week-old wild-type ( c ) or Tgr5 −/− ( d ) mice treated by gavage for 5 days with GW4064 (30 mpk; n =5 mice per group. Data are represented as mean ±s.d. ( e ) Proglucagon qPCR on cDNA from isolated primary intestinal epithelial cells from two wild-type mice ex vivo treated for 24 h with DMSO or with GW4064 (5 μmol l −1 ). ( f ) Proglucagon qPCR on cDNA of human jejunal biopsies from four normoglycemic patients ex vivo treated for 16 h with DMSO or with GW4064 (5 μmol l −1 ). Data are represented as mean ±−s.e.m. Student’s t -test, * P ≤0.05, ** P ≤0.01 and *** P ≤0.001. Full size image To assess whether FXR activation controls the production of GLP-1, one of the major bio-active peptides produced by L cells, 8-week-old C57Bl6-J wild-type mice were daily treated by gavage with the FXR agonist GW4064 (30 mpk) for 5 days. As expected Fgf15 mRNA levels increase after FXR agonist treatment ( Supplementary Fig. 1b ), whereas proglucagon mRNA levels decrease in both the ileum and colon ( Fig. 1c ). Since treatment with GW4064 modulates the bile acid pool composition leading to lower amount of TGR5 activators [13] , proglucagon mRNA levels were measured in intestines of Tgr5−/− mice treated during 5 days with GW4064 (30 mpk). FXR activation significantly decreases proglucagon mRNA levels in the ileum of Tgr5−/− mice and to a lesser extent in the colon, suggesting a crosstalk between FXR and TGR5 in the colon, but not the ileum ( Fig. 1d ). This finding is consistent with elevated levels of secondary BA that activate TGR5 in the colon. In addition, primary murine intestinal epithelial cells treated ex vivo with GW4064 (5 μmol l −1 ) also exhibited decreased proglucagon mRNA levels ( Fig. 1e ) showing that in addition to changes in bile acid pool composition, FXR activation directly decreases proglucagon gene expression. As FXR is also expressed in human intestinal L cells ( Fig. 1b ), human jejunal biopsies were treated with GW4064 (5 μmol l −1 ). FXR activation results in the expected induction of mRNA levels of FGF19 , the human FGF15 orthologue ( Supplementary Fig. 1c ), whereas proglucagon gene expression decreases ( Fig. 1f ). FXR activation decreases proglucagon expression in vitro To study the mechanisms underlying the regulation of proglucagon gene expression by FXR, the well-characterized murine L-cell model GLUTag was used [26] , [27] . FXR mRNA ( Fxr Ct=28; cyclophilin Ct=22) and protein are expressed and enriched in the nuclear fraction ( Fig. 2a ). Moreover, incubation of GLUTag cells with increasing concentrations of GW4064 results in the induction of the FXR target genes Shp ( Fig. 2b ) and Fgf15 ( Fig. 2c ). Similar as in human and murine hepatocytes [11] , [28] , GW4064 treatment (5 μmol l −1 ) increases FXR mRNA and protein expression, whereas siRNA knockdown of FXR decreases >50% FXR mRNA ( Fig. 2d ) and protein levels ( Fig. 2e ). The induction of Fgf15 by GW4064 decreases by 10-fold in si Fxr -transfected GLUTag cells ( Fig. 2f ). Altogether, these data indicate the presence of functional FXR in GLUTag cells. 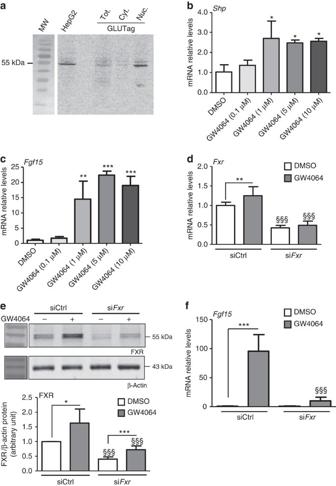Figure 2: FXR is expressed and functional in GLUTag L cells. (a) Representative western blot of four experiments performed with fractioned protein extracts from GLUTag cells. Total proteins from HepG2 are used as control.Shp(b) andFgf15(c) qPCRs on cDNA from GLUTag cells treated for 24 h with GW4064 (0.1, 1, 5 and 10 μmol l−1). Data are represented as mean ± s.d. One-way analysis of variance (ANOVA) followed by Tukey’spost hoctest. *P≤0.05, **P≤0.01 and ***P≤0.001 versus DMSO (n=3; performed three times). (d)FxrqPCR on cDNA from GLUTag cells electroporated with siCtrl or siFxrand treated for 24 h with GW4064 (5 μmol l−1;n=3; performed three times). (e) Representative western blot of four experiments performed on protein extracts from GLUTag cells electroporated with a siCtrl or with a siFxrand treated for 24 h with GW4064 (5 μmol l−1; upper panel) and quantification (lower panel) of FXR from four western blots (n=3). (f)Fgf15qPCR on cDNA from GLUTag cells electroporated with siCtrl or siFxrand treated for 24 h with GW4064 (5 μmol l−1;n=3; performed three times). Data are represented as mean ± s.d. Two-way ANOVA analysis followed by Bonferronni’spost hoctest. *P≤0.05, **P≤0.01 and ***P≤0.001 versus DMSO of transfection-matched condition and§§§P≤0.001 versus siCtrl of treatment-matched condition. Figure 2: FXR is expressed and functional in GLUTag L cells. ( a ) Representative western blot of four experiments performed with fractioned protein extracts from GLUTag cells. Total proteins from HepG2 are used as control. Shp ( b ) and Fgf15 ( c ) qPCRs on cDNA from GLUTag cells treated for 24 h with GW4064 (0.1, 1, 5 and 10 μmol l −1 ). Data are represented as mean ± s.d. One-way analysis of variance (ANOVA) followed by Tukey’s post hoc test. * P ≤0.05, ** P ≤0.01 and *** P ≤0.001 versus DMSO ( n =3; performed three times). ( d ) Fxr qPCR on cDNA from GLUTag cells electroporated with siCtrl or si Fxr and treated for 24 h with GW4064 (5 μmol l −1 ; n =3; performed three times). ( e ) Representative western blot of four experiments performed on protein extracts from GLUTag cells electroporated with a siCtrl or with a si Fxr and treated for 24 h with GW4064 (5 μmol l −1 ; upper panel) and quantification (lower panel) of FXR from four western blots ( n =3). ( f ) Fgf15 qPCR on cDNA from GLUTag cells electroporated with siCtrl or si Fxr and treated for 24 h with GW4064 (5 μmol l −1 ; n =3; performed three times). Data are represented as mean ± s.d. Two-way ANOVA analysis followed by Bonferronni’s post hoc test. * P ≤0.05, ** P ≤0.01 and *** P ≤0.001 versus DMSO of transfection-matched condition and §§§ P ≤0.001 versus siCtrl of treatment-matched condition. Full size image Incubation of GLUTag cells for 24 h with increasing concentrations of GW4064 or with GW4064 (5 μmol l −1 ) for different times in standard culture glucose concentrations (5.6 mmol l −1 ) decreases proglucagon mRNA levels in a dose- and time-dependent manner with a maximum effect at 5 μmol l −1 ( Fig. 3a ), a concentration often used to study FXR activation [12] , [28] , after 24 h of treatment ( Fig. 3b ). Moreover, a similar decrease is observed with the natural FXR ligand chenodeoxycholic acid (CDCA, 100 μmol l −1 ) ( Supplementary Fig. 2a ). Using primer combination covering exon 2 to intron 2 of the proglucagon gene, a similar decrease of proglucagon pre-mRNA levels is observed, suggesting that FXR negatively regulates proglucagon gene transcription ( Supplementary Fig. 2b ). GW4064 incubation decreases proglucagon mRNA and protein levels in siCtrl cells, whereas such a decrease is not observed in si Fxr cells, indicating that FXR is required for the decrease of proglucagon gene expression upon GW4064 treatment ( Fig. 3c,d ). 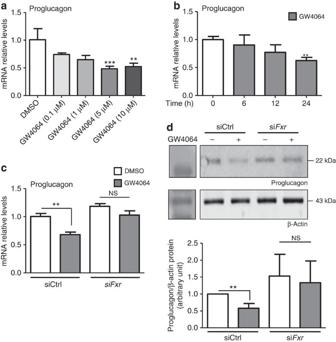Figure 3: FXR activation decreases proglucagon mRNA in GLUTag cells. (a) Proglucagon qPCR on cDNA from GLUTag cells treated for 24 h with GW4064 (0.1, 1, 5 or 10 μmol l−1;n=3; performed three times). Data are represented as mean ± s.d. One-way analysis of variance (ANOVA) followed by Tukey’spost hoctest. **P≤0.01 and ***P≤0.001 versus DMSO. (b) Proglucagon qPCR on cDNA from GLUTag cells treated for 0, 6, 12 or 24 h with GW4064 (5 μmol l−1;n=3; performed three times). Data are represented as mean ± s.d. One-way ANOVA followed by Tukey’spost hoctest. **P≤0.01 versus t0. (c) Proglucagon qPCR on cDNA from GLUTag cells electroporated with siCtrl or siFxrand treated for 24 h with GW4064 (5 μmol l−1). (d) Representative western blot of four experiments performed on protein extracts from GLUTag cells electroporated with a siCtrl or with a siFxrand treated for 24 h with GW4064 (5 μmol l−1; upper panel) and quantification (lower panel) of proglucagon from four western blots (n=3). Data are represented as mean ±s.d. Two-way ANOVA analysis followed by Bonferronni’spost hoctest. **P≤0.01: effect of GW4064 in each transfection condition. Figure 3: FXR activation decreases proglucagon mRNA in GLUTag cells. ( a ) Proglucagon qPCR on cDNA from GLUTag cells treated for 24 h with GW4064 (0.1, 1, 5 or 10 μmol l −1 ; n =3; performed three times). Data are represented as mean ± s.d. One-way analysis of variance (ANOVA) followed by Tukey’s post hoc test. ** P ≤0.01 and *** P ≤0.001 versus DMSO. ( b ) Proglucagon qPCR on cDNA from GLUTag cells treated for 0, 6, 12 or 24 h with GW4064 (5 μmol l −1 ; n =3; performed three times). Data are represented as mean ± s.d. One-way ANOVA followed by Tukey’s post hoc test. ** P ≤0.01 versus t0. ( c ) Proglucagon qPCR on cDNA from GLUTag cells electroporated with siCtrl or si Fxr and treated for 24 h with GW4064 (5 μmol l −1 ). ( d ) Representative western blot of four experiments performed on protein extracts from GLUTag cells electroporated with a siCtrl or with a si Fxr and treated for 24 h with GW4064 (5 μmol l −1 ; upper panel) and quantification (lower panel) of proglucagon from four western blots ( n =3). Data are represented as mean ±s.d. Two-way ANOVA analysis followed by Bonferronni’s post hoc test. ** P ≤0.01: effect of GW4064 in each transfection condition. Full size image FXR inhibits glucose-induced proglucagon expression It has previously been shown that glucose induces proglucagon gene expression in GLUTag L cells [26] . Moreover, in hepatocytes, FXR activation inhibits the induction of glycolytic and lipogenic genes by glucose [12] . To determine whether FXR activation also inhibits the glucose response in L cells, GLUTag cells were cultured for 12 h in glucose-free medium and subsequently incubated in medium containing lactate (10 mmol l −1 ), glucose (5.6 mmol l −1 ) or 2-deoxyglucose (5.6 mmol l −1 ; Fig. 4a ). As expected [26] , glucose increases proglucagon gene expression ( Fig. 4a ). 2-Deoxyglucose, a non-metabolised glucose analogue, does not increase proglucagon mRNA levels, highlighting that glucose metabolism is mandatory for the glucose-induced proglucagon gene expression. Moreover, FXR activation for 24 h with either GW4064 or CDCA inhibits proglucagon gene expression only in L cells incubated in standard (5.6 mmol l −1 ), but not in low glucose concentrations ( Fig. 4a ). 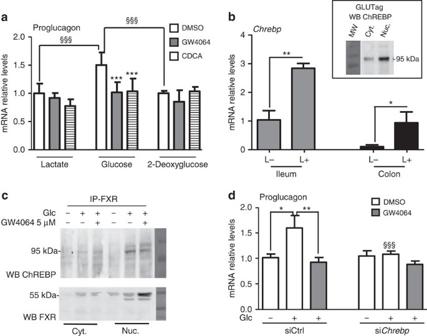Figure 4: FXR inhibits glucose-induced proglucagon expression. (a) Proglucagon qPCR on cDNA from GLUTag cells starved for 12 h with lactate (10 mmol l−1) and then incubated for 24 h in lactate (10 mmol l−1), glucose (5.6 mmol l−1) or 2-deoxyglucose (5.6 mmol l−1) media containing DMSO, GW4064 (5 μmol l−1) or CDCA (100 μmol l−1;n=3; performed three times). Data are represented as mean ±s.d. Two-way analysis of variance (ANOVA) followed by Bonferronni’spost hoctest. ***P≤0.001: effect of GW4064 and CDCA on proglucagon mRNA levels in each medium conditions.§§§P≤0.001: effect of glucose on proglucagon mRNA levels in DMSO, GW4064 and CDCA conditions. (b)ChrebpqPCR on cDNA from FACS-sorted proglucagon-negative and proglucagon-positive cells from the ileum (ileum L−; ileum L+) and colon (colon L−; colon L+) of GLU-VENUS mice (lower panel;n=3) and ChREBP protein expression from cytoplasm and nucleus extract from GLUTag cells (upper panel; performed three times). Data are represented as mean ±s.d. Student’st-test. *P≤0.05 and **P≤0.01 (c) ChREBP and FXR western blots after FXR immunoprecipitation on lysates from cytoplasm and nucleus of GLUTag cells treated or not with GW4064 (5 μmol l−1) in the presence or not of glucose (5.6 mmol l−1; performed two times). (d) Proglucagon qPCR on cDNA from GLUTag cells electroporated with a siCtrl or siChrebp, starved for 12 h with lactate (10 mmol l−1) and then incubated for 24 h in lactate 10 mmol l−1(Glc−) or glucose 5.6 mmol l−1(Glc+) media supplemented with DMSO or GW4064 (5 μmol l−1;n=3; performed three times). Data are represented as mean ±s.d. Two-way ANOVA analysis followed by Bonferronni’spost hoctest. *P≤0.05 and **P≤0.01: effect of treatments on each transfection condition.§§§P≤0.001: effect of siChrebpin each treatment condition. Figure 4: FXR inhibits glucose-induced proglucagon expression. ( a ) Proglucagon qPCR on cDNA from GLUTag cells starved for 12 h with lactate (10 mmol l −1 ) and then incubated for 24 h in lactate (10 mmol l −1 ), glucose (5.6 mmol l −1 ) or 2-deoxyglucose (5.6 mmol l −1 ) media containing DMSO, GW4064 (5 μmol l −1 ) or CDCA (100 μmol l −1 ; n =3; performed three times). Data are represented as mean ±s.d. Two-way analysis of variance (ANOVA) followed by Bonferronni’s post hoc test. *** P ≤0.001: effect of GW4064 and CDCA on proglucagon mRNA levels in each medium conditions. §§§ P ≤0.001: effect of glucose on proglucagon mRNA levels in DMSO, GW4064 and CDCA conditions. ( b ) Chrebp qPCR on cDNA from FACS-sorted proglucagon-negative and proglucagon-positive cells from the ileum (ileum L−; ileum L+) and colon (colon L−; colon L+) of GLU-VENUS mice (lower panel; n =3) and ChREBP protein expression from cytoplasm and nucleus extract from GLUTag cells (upper panel; performed three times). Data are represented as mean ±s.d. Student’s t -test. * P ≤0.05 and ** P ≤0.01 ( c ) ChREBP and FXR western blots after FXR immunoprecipitation on lysates from cytoplasm and nucleus of GLUTag cells treated or not with GW4064 (5 μmol l −1 ) in the presence or not of glucose (5.6 mmol l −1 ; performed two times). ( d ) Proglucagon qPCR on cDNA from GLUTag cells electroporated with a siCtrl or si Chrebp , starved for 12 h with lactate (10 mmol l −1 ) and then incubated for 24 h in lactate 10 mmol l −1 (Glc−) or glucose 5.6 mmol l −1 (Glc+) media supplemented with DMSO or GW4064 (5 μmol l −1 ; n =3; performed three times). Data are represented as mean ±s.d. Two-way ANOVA analysis followed by Bonferronni’s post hoc test. * P ≤0.05 and ** P ≤0.01: effect of treatments on each transfection condition. §§§ P ≤0.001: effect of si Chrebp in each treatment condition. Full size image As ChREBP is a glucose-sensitive transcription factor activated by glucose metabolites [29] and since FXR activation interferes with the ChREBP-mediated induction of glycolytic enzyme gene expression by glucose in hepatocytes [12] , we next assessed whether this regulatory mechanism is operational also in L cells. Using L cells isolated from GLU-VENUS mice, ChREBP is found to be expressed at higher levels in L cells than in non-L cells ( Fig. 4b ). Moreover, ChREBP is also expressed in GLUTag L-cells ( Fig. 4b insert). FXR immunoprecipitation from cytoplasmic and nuclear protein fractions demonstrates that ChREBP and FXR physically interact or are in the same complexes in high glucose conditions ( Fig. 4c ), similar as in hepatocytes [12] . Finally, siRNA knockdown of ChREBP, resulting in ≥50% decrease of Chrebp mRNA levels ( Supplementary Fig. 3 ), prevents the induction of proglucagon mRNA levels by glucose ( Fig. 4d ). FXR activation by GW4064 inhibits the increase of proglucagon mRNA levels by glucose in siCtrl transfected cells, whereas this effect is not observed in ChREBP knockdown cells. Taken together, these data demonstrate that glucose metabolism through the glycolysis pathway is necessary for the glucose-dependent ChREBP-mediated increase of proglucagon gene expression, which is inhibited upon FXR activation. FXR decreases glycolysis and glucose-induced GLP-1 secretion GLP-1 secretion in response to glucose occurs, at least in part, through glucose metabolism by glycolysis [24] , [30] , [31] . DNA microarray followed by Gene Ontology analysis was performed on GW4064-treated GLUTag cells. Interestingly, GW4064 treatment downregulates the expression of several glycolytic genes leading to a significant inhibition of this pathway ( P =4.33 × 10 −6 ; Fig. 5a ). This decrease translates into lower basal and glucose-enhanced intracellular ATP levels ( Fig. 5b ). GW4064 treatment does not decrease mitochondrial mass as assessed by the Mitotracker Green assay ( Fig. 5c ). However, glycolytic capacity assessed by measurement of the extracellular acidification rate (ECAR) after oligomycin treatment is lower in GW4064 pre-treated cells ( Fig. 5d ). In parallel, FXR activation decreases basal- and ATP-dependent oxygen consumption rates (OCR) in GW4064-treated cells ( Supplementary Fig. 4 ) likely reflecting the decrease in activity of the global glycolysis pathway as also suggested by the microarray results. Finally, FXR activation results in lower basal and glucose-induced GLP-1 secretion ( Fig. 5e ). As GW4064 does not modulate KCl-induced GLP-1 secretion ( Fig. 5e ), it is unlikely that FXR modulates electrogenic events and that its action occurs rather upstream of membrane depolarization. Even though initial reports suggested that the SGLT-1/electrogenic pathway is the main mechanism by which glucose induces GLP-1 secretion in primary intestinal epithelial cells [24] , [27] , recent observations on perfused rat ileums indicate that, in addition to the SGLT-1 pathway, the glucose metabolism-mediated pathway contributes to the full GLP-1 secretion response to glucose [30] , [31] . Therefore, the response to glucose (5.6 mmol l −1 ) with or without the GLUTs inhibitor phloretin on GLP-1 secretion in murine ileal biopsies was tested. Glucose alone induces GLP-1 secretion by tissue explants from vehicle-treated mice, whereas co-incubation with phloretin completely blocked the glucose response ( Fig. 5f ). Moreover, in vivo GW4064 treatment (5 days, 30 mpk) prevents the increase in glucose-induced GLP-1 secretion by the ileum ex vivo ( Fig. 5f ), but is without effect in the presence of phloretin ( Fig. 5f ), indicating that glucose transport by the GLUT-transporter appears mandatory for the inhibitory effect of FXR activation on the GLP-1 response to glucose. 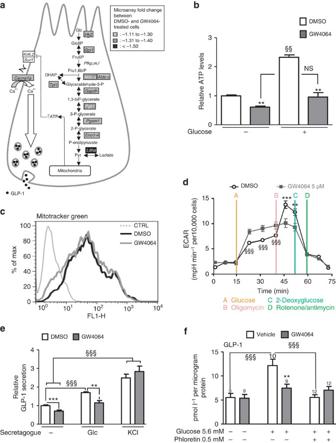Figure 5: FXR inhibits GLP-1 secretion by decreasing glycolysis. (a) DNA microarrays on 24 h DMSO- and GW4064(5 μmol l−1)-treated GLUTag cells were performed using Agilent Technology. Genes whose expression is downregulated by 10%, 10%− 30% and upregulated by 50% after GW4064 treatment are written with black letters in rectangles filled in grey, with white letters in rectangles filled in grey and with white letters in black filled rectangles, respectively.Pvalue of the glycolysis biological process:P=4.33 × 10−6. (b) ATP measurements on GLUTag cells treated for 24 h with GW4064(5 μmol l−1) and stimulated or not for 1 h with glucose(5.6 mmol l−1).§§P≤0.01: effect of glucose on ATP levels. **P≤0.01: effect of GW4064 on ATP levels. (c) Fluorescence measurements by Mitotracker Green in GLUTag cells incubated with DMSO or GW4064 (n=3; performed three times). (d) Extracellular acidification rate (ECAR) after successive injection of glucose(10 mmol l−1), oligomycin(1 μmol l−1), 2-deoxyglucose(100 mmol l−1) and rotenone(1 μmol l−1)/antimycin A(1 μmol l−1) on GLUTag cells incubated 24 h with DMSO or GW4064.§§§P≤0.001: effect of GW4064 on ECAR betweent=15 min andt=40 min. **P≤0.01 and ***P≤0.001: effect of GW4064 on ECAR betweent=40 min andt=55 min. Representative results of four independent experiments. (e) GLP-1 measurements in supernatants of GLUTag cells treated for 24 h with GW4064(5 μmol l−1) and stimulated or not for 1 h with 5.6 mmol l−1of glucose- or 30 mmol l−1of KCl-containing buffer (n=3; performed four times). **P≤0.01, ***P≤0.001: effect of GW4064 treatment in each secretion condition.§§§P≤0.001: effect of secretagogue in each treatment condition. (f) GLP-1 measurements in supernatants of intestinal biopsies from WT mice treated for 5 days with vehicle or with GW4064(30 mpk) and then stimulated with medium alone, medium plus glucose(5.6 mM) or medium plus glucose(5.6 mol l−1) plus phloretin(0.5 mmol l−1). **P≤0.01: effect of GW4064 treatment on GLP-1 secretion in each secretion condition.§§§P≤0.001: effect of secretagogues on each treatment condition. On the bars, number of biopsies used from three vehicle- or GW4064 (30 mpk)-treated mice. Data are represented as mean ±s.d. (b,dande) or mean±s.e.m. (f). Statistical analysis were performed using two-way analysis of variance followed by Bonferronni’spost hoctest. Figure 5: FXR inhibits GLP-1 secretion by decreasing glycolysis. ( a ) DNA microarrays on 24 h DMSO- and GW4064(5 μmol l −1 )-treated GLUTag cells were performed using Agilent Technology. Genes whose expression is downregulated by 10%, 10%− 30% and upregulated by 50% after GW4064 treatment are written with black letters in rectangles filled in grey, with white letters in rectangles filled in grey and with white letters in black filled rectangles, respectively. P value of the glycolysis biological process: P =4.33 × 10 −6 . ( b ) ATP measurements on GLUTag cells treated for 24 h with GW4064(5 μmol l −1 ) and stimulated or not for 1 h with glucose(5.6 mmol l −1 ). §§ P ≤0.01: effect of glucose on ATP levels. ** P ≤0.01: effect of GW4064 on ATP levels. ( c ) Fluorescence measurements by Mitotracker Green in GLUTag cells incubated with DMSO or GW4064 ( n =3; performed three times). ( d ) Extracellular acidification rate (ECAR) after successive injection of glucose(10 mmol l −1 ), oligomycin(1 μmol l −1 ), 2-deoxyglucose(100 mmol l −1 ) and rotenone(1 μmol l −1 )/antimycin A(1 μmol l −1 ) on GLUTag cells incubated 24 h with DMSO or GW4064. §§§ P ≤0.001: effect of GW4064 on ECAR between t =15 min and t =40 min. ** P ≤0.01 and *** P ≤0.001: effect of GW4064 on ECAR between t =40 min and t =55 min. Representative results of four independent experiments. ( e ) GLP-1 measurements in supernatants of GLUTag cells treated for 24 h with GW4064(5 μmol l −1 ) and stimulated or not for 1 h with 5.6 mmol l −1 of glucose- or 30 mmol l −1 of KCl-containing buffer ( n =3; performed four times). ** P ≤0.01, *** P ≤0.001: effect of GW4064 treatment in each secretion condition. §§§ P ≤0.001: effect of secretagogue in each treatment condition. ( f ) GLP-1 measurements in supernatants of intestinal biopsies from WT mice treated for 5 days with vehicle or with GW4064(30 mpk) and then stimulated with medium alone, medium plus glucose(5.6 mM) or medium plus glucose(5.6 mol l −1 ) plus phloretin(0.5 mmol l −1 ). ** P ≤0.01: effect of GW4064 treatment on GLP-1 secretion in each secretion condition. §§§ P ≤0.001: effect of secretagogues on each treatment condition. On the bars, number of biopsies used from three vehicle- or GW4064 (30 mpk)-treated mice. Data are represented as mean ±s.d. ( b , d and e ) or mean±s.e.m. ( f ). Statistical analysis were performed using two-way analysis of variance followed by Bonferronni’s post hoc test. Full size image Taken together, these data show that FXR activation decreases the glycolysis pathway leading to decreased ATP levels and a lower GLP-1 secretion in response to glucose. Fxr deficiency increases proglucagon mRNA and GLP-1 levels FXR-deficient mice display elevated proglucagon mRNA levels in the ileum and colon ( Fig. 6a ) and enhanced active GLP-1 plasma concentrations 15 min after oral glucose administration ( Fig. 6b ). Since conventionally raised (CONV-R) and GF mice display different FXR antagonist:agonist ratios leading to FXR inhibition in GF mice [17] , proglucagon mRNA levels were compared in CONV-R and GF WT and FXR-deficient mice. As expected [17] , Fgf15 gene expression is repressed in GF compared with CONV-R mice, similar to that in Fxr−/− mice ( Fig. 6c ). Moreover, CONV-R Fxr−/− mice display higher proglucagon mRNA levels compared with CONV-R Fxr+/+ mice ( Fig. 6d ), whereas in GF mice, FXR deficiency no further modulates proglucagon mRNA levels ( Fig. 6d ). In vitro incubation of GLUTag cells with TβMCA (100 μmol l −1 ) decreases Fgf15 gene expression ( Fig. 6e ) and increases proglucagon gene expression ( Fig. 6f ), suggesting a crosstalk between BA, FXR and microbiota in the regulation of proglucagon gene expression in L cells. 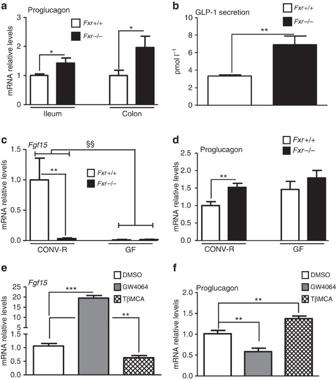Figure 6:Fxr−/−mice exhibit higher proglucagon mRNA and GLP-1 levels. (a) Proglucagon qPCR on cDNA from ileum and colon of 8-week-oldFxr+/+orFxr−/−mice.n=5–6 mice per group. (b) GLP-1 secretion in 8-week-oldFxr+/+orFxr−/−mice 15 min after an oral challenge with glucose 2 g kg−1.n=5–6 mice per group. Data are represented as mean ±s.e.m. Student’st-test, *P≤0.05 and **P≤0.01.Fgf15(c) and Proglucagon (d) qPCR on cDNA from ileum of 8-week-old GF or CONV-R mice on aFxr+/+or aFxr−/−background (n=11–12 mice per group). Data are represented as mean ±s.e.m. Two-way analysis of variance (ANOVA) followed by Bonferronni’spost hoctest. **P≤0.01: effect of FXR deficiency on gene expression in each raised condition.§§P≤0.01: effect of gut microbiota on gene expression in each genotype.Fgf15(e) and Proglucagon (f) qPCR on cDNA from GLUTag cells treated for 24 h with GW4064 (5 μmol l−1) or with TβMCA (100 μmol l−1;n=3; performed three times). Data are represented as mean ±s.d. One-way ANOVA followed by Tukey’spost hoctest. **P≤0.01, ***P≤0.001 versus DMSO. Figure 6: Fxr−/− mice exhibit higher proglucagon mRNA and GLP-1 levels. ( a ) Proglucagon qPCR on cDNA from ileum and colon of 8-week-old Fxr+/+ or Fxr−/− mice. n =5–6 mice per group. ( b ) GLP-1 secretion in 8-week-old Fxr+/+ or Fxr−/− mice 15 min after an oral challenge with glucose 2 g kg −1 . n =5–6 mice per group. Data are represented as mean ±s.e.m. Student’s t -test, * P ≤0.05 and ** P ≤0.01. Fgf15 ( c ) and Proglucagon ( d ) qPCR on cDNA from ileum of 8-week-old GF or CONV-R mice on a Fxr+/+ or a Fxr−/− background ( n =11–12 mice per group). Data are represented as mean ±s.e.m. Two-way analysis of variance (ANOVA) followed by Bonferronni’s post hoc test. ** P ≤0.01: effect of FXR deficiency on gene expression in each raised condition. §§ P ≤0.01: effect of gut microbiota on gene expression in each genotype. Fgf15 ( e ) and Proglucagon ( f ) qPCR on cDNA from GLUTag cells treated for 24 h with GW4064 (5 μmol l −1 ) or with TβMCA (100 μmol l −1 ; n =3; performed three times). Data are represented as mean ±s.d. One-way ANOVA followed by Tukey’s post hoc test. ** P ≤0.01, *** P ≤0.001 versus DMSO. Full size image Thus, modulation of endogenous FXR ligands by the microbiota may influence proglucagon gene expression in an FXR-dependent manner. FXR deficiency improves glycaemia through the GLP-1R pathway It is well known that FXR deficiency protects mice against diet-induced obesity and improves glucose homeostasis [14] , [32] , [33] . To test the metabolic impact of the FXR/GLP-1 pathway in a pathophysiological context, Fxr+/+ and Fxr−/− mice were fed a high-fat diet (HFD) during 6 weeks before metabolic tests with or without the GLP-1R antagonist Exendin-4(9-39). After 6 weeks of diet, Fxr+/+ mice gain 44% of their initial body mass, whereas, as expected [14] , [32] , [33] , high-fat-fed Fxr−/− mice only gain 23%. Intraperitoneal GTT (2 g kg −1 ) reveals only a minor, nonsignificant decrease in glucose excursion curve in Fxr−/− versus Fxr+/+ mice ( Fig. 7a ). However, when challenged with an oral glucose bolus (2 g kg −1 ), Fxr−/− mice display an improved glucose tolerance compared with Fxr+/+ mice (45% decrease in integrated area under the curve (iAUC), P ≤0.05, Fig. 7b ) reflecting a role of the intestine in the regulation of glucose homeostasis by FXR. To assess the involvement of the GLP-1 pathway in this improvement, the GLP-1R antagonist Exendin-4(9-39) was administered before the oral glucose gavage test. Glucose tolerance worsens in Exendin-4(9-39)-treated mice of both genotypes ( Fig. 7b–d ) with a more pronounced effect in Fxr−/− mice ( Fig. 7b , +30% in iAUC in Fxr+/+ versus +80% in iAUC in Fxr−/− mice), hence abolishing the beneficial effect on oral glucose tolerance of FXR deficiency. 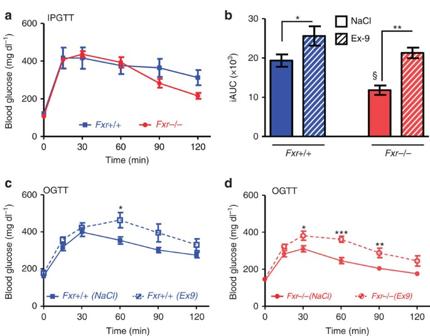Figure 7: FXR deficiency improves glucose metabolism via the GLP-1 pathway. (a) Intraperitoneal glucose tolerance test in 12-week-oldFxr+/+andFxr−/−mice fed for 6 weeks with a 60% HFD (n=6 mice per group). Data are represented as mean ±s.e.m. (b) Integrated area under the curve (iAUC) of glucose excursion curves after 0.9% NaCl or Exendin-4(9-39) (0.5 mpk) injection 45 min before an oral glucose tolerance test (OGTT, 2 g kg−1) inFxr+/+andFxr−/−mice fed for 6 weeks with a 60% HFD (n=6 mice per group). Data are represented as mean ±s.e.m. Two-way analysis of variance (ANOVA) followed by Bonferronni’spost hoctest. *P≤0.05 and **P≤0.01: effect of Exendin-4(9-39) on iAUC in each genotype.§P≤0.05: effect of genotype in each treatment condition. OGTT after 0.9% NaCl or Exendin-4(9-39) (0.5 mpk) in 12-week-oldFxr+/+(c) andFxr−/−(d) mice fed for 6 weeks with a HFD 60% (n=6 mice per group). Data are represented as mean ±s.e.m. Two-way ANOVA analysis followed by Bonferronni’spost hoctest. *P≤0.05, **P≤0.01 and ***P≤0.001: effect of Exendin-4(9-39) treatment on glucose excursion in each genotype. Figure 7: FXR deficiency improves glucose metabolism via the GLP-1 pathway. ( a ) Intraperitoneal glucose tolerance test in 12-week-old Fxr+/+ and Fxr−/− mice fed for 6 weeks with a 60% HFD ( n =6 mice per group). Data are represented as mean ±s.e.m. ( b ) Integrated area under the curve (iAUC) of glucose excursion curves after 0.9% NaCl or Exendin-4(9-39) (0.5 mpk) injection 45 min before an oral glucose tolerance test (OGTT, 2 g kg −1 ) in Fxr+/+ and Fxr−/− mice fed for 6 weeks with a 60% HFD ( n =6 mice per group). Data are represented as mean ±s.e.m. Two-way analysis of variance (ANOVA) followed by Bonferronni’s post hoc test. * P ≤0.05 and ** P ≤0.01: effect of Exendin-4(9-39) on iAUC in each genotype. § P ≤0.05: effect of genotype in each treatment condition. OGTT after 0.9% NaCl or Exendin-4(9-39) (0.5 mpk) in 12-week-old Fxr+/+ ( c ) and Fxr−/− ( d ) mice fed for 6 weeks with a HFD 60% ( n =6 mice per group). Data are represented as mean ±s.e.m. Two-way ANOVA analysis followed by Bonferronni’s post hoc test. * P ≤0.05, ** P ≤0.01 and *** P ≤0.001: effect of Exendin-4(9-39) treatment on glucose excursion in each genotype. Full size image These results show that the GLP-1/GLP-1R pathway contributes to the improved glucose homeostasis upon FXR deficiency. BAS improve glycaemia and GLP-1 production by FXR To test the response to pharmacological targeting of the FXR/GLP-1 pathway, ob/ob Fxr+/+ and ob/ob Fxr−/− mice were treated for 2 weeks with colesevelam, a BAS known to deactivate intestinal FXR [23] . As expected, BAS administration inhibits FXR activity in the ileum and colon as reflected by repression of Fgf15 gene expression ( Supplementary Fig. 5a,b ). BAS improves glucose metabolism after an OGTT in ob/ob Fxr+/+ mice, an effect not observed in ob/ob Fxr−/− mice ( Fig. 8a–c ). Moreover, BAS administration increases proglucagon gene expression in the ileum ( Fig. 8d ) and colon ( Supplementary Fig. 5c ) only in ob/ob Fxr+/+ mice, an effect which may contribute to the improved glucose control. 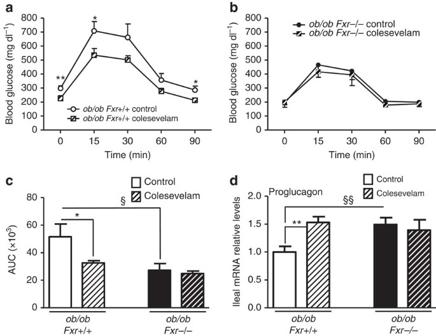Figure 8: BA sequestration improves glycaemia and GLP-1 production through FXR. OGTT after 3 weeks of vehicle or colesevelam treatment inob/ob Fxr+/+(a) andob/ob Fxr−/−mice (b) (n=6–7 mice per group). (c) Corresponding area under the curve (AUC). (d) Proglucagon qPCR on cDNA from ileum of these mice (n=6–7 mice per group). Data are represented as mean ±s.e.m. Two-way analysis of variance (ANOVA) followed by Bonferronni’spost hoctest. *P≤0.05 and **P≤0.01: effect of Colesevelam treatment on glucose excursion curve during an OGTT (aandb), on AUC (c) or on proglucagon gene expression (d) in each genotype.§P≤0.05,§§P≤0.01: effect of FXR deficiency on AUC (c) or on proglucagon gene expression (d) in each treatment condition. Figure 8: BA sequestration improves glycaemia and GLP-1 production through FXR. OGTT after 3 weeks of vehicle or colesevelam treatment in ob/ob Fxr+/+ ( a ) and ob/ob Fxr−/− mice ( b ) ( n =6–7 mice per group). ( c ) Corresponding area under the curve (AUC). ( d ) Proglucagon qPCR on cDNA from ileum of these mice ( n =6–7 mice per group). Data are represented as mean ±s.e.m. Two-way analysis of variance (ANOVA) followed by Bonferronni’s post hoc test. * P ≤0.05 and ** P ≤0.01: effect of Colesevelam treatment on glucose excursion curve during an OGTT ( a and b ), on AUC ( c ) or on proglucagon gene expression ( d ) in each genotype. § P ≤0.05, §§ P ≤0.01: effect of FXR deficiency on AUC ( c ) or on proglucagon gene expression ( d ) in each treatment condition. Full size image Using transgenic VENUS mice expressing the reporter gene only in proglucagon-positive cells and human biopsies, we show that FXR is not only expressed in the enterocyte but also in L cells, where its activity was demonstrated by agonist-induced regulation of two bona fide FXR target genes, Fgf15 and Shp . Both in vitro , ex vivo and in vivo , in mice as well as in human intestines, activated FXR decreases proglucagon mRNA levels. This decrease is the result of FXR activation in L cells rather than an indirect effect of bile acid pool modification after FXR activation. ChREBP is a transcription factor activated by glucose metabolites. As previously evoked by microarray data [25] , we demonstrate by quantitative PCR (qPCR) analysis that ChREBP is expressed to a higher extent in murine intestinal L cells than in non-L cells. Moreover, glucose induction of proglucagon mRNA levels [26] is inhibited by FXR activation. We identify here that glucose-induced proglucagon gene expression is dependent on glucose metabolism and mediated by ChREBP, identifying a role for ChREBP in enteroendocrine L cells in the control of proglucagon gene expression. FXR physically interacts or is complexed to ChREBP in L cells, a result also observed in human hepatocytes where FXR activation inhibits the glucose-induced glycolytic gene expression by ChREBP [12] . These observations are in accordance with an overall decrease of the glycolysis pathway after FXR activation in GLUTag cells similar to that in human hepatocytes. Glucose sensing by L cells and subsequent secretion of GLP-1 involves both ATP-independent and -dependent pathways [24] , [30] , [31] . The ATP-independent mechanism is mediated by the co-transport of Na + and glucose through the membrane transporter SGLT-1 (refs 27 , 31 , 34 , 35 ) and glucose binding to the taste receptors Tas1R2 and Tas1R3 (ref. 36 ). The electrogenic current generated by the Na + entrance is sufficient to depolarize L-cell membranes leading to GLP-1 secretion. This mechanism has been shown to be involved in glucose-induced GLP-1 secretion in GLUTag cells, in perfused rat ileum and also in primary intestinal epithelial cells [24] , [27] , [31] , [34] . The ATP-dependent pathway involves glucose metabolism by glycolysis, thus increasing intracellular ATP levels, closure of the voltage-dependent K ATP -dependent channel, membrane depolarization, intracellular Ca 2+ increase and GLP-1 secretion. Such a mechanism is involved in glucose-induced GLP-1 secretion in GLUTag cells [27] , in perfused rat ileum [31] but not in primary intestinal epithelial cells [27] . We show that FXR activation does not decrease the expression of Sglt1 , Tas1r2 , Tas1r3 in GLUTag cells. Moreover, FXR activation did not change KCl-induced GLP-1 secretion, but lowered GLP-1 secretion in response to both low and high glucose concentrations. Glucose transport by GLUT transporters is required for intracellular ATP production in L cells [24] . Indeed, incubation of murine intestinal biopsies with the GLUTs inhibitor phloretin prevented glucose-induced GLP-1 secretion. FXR activation prevented glucose-induced GLP-1 secretion in isolated murine ileal biopsies to a similar extent as phloretin. To delineate the mechanisms underlying the decrease of ATP-dependent GLP-1 secretion by FXR, we assessed the activity of the glycolysis pathway and the functionality of mitochondria in GLUTag cells. FXR activation decreased intracellular ATP levels, independent of a decrease in mitochondrial mass or defective mitochondria, as seen with Mitotracker Green and OCR experiments. ECAR measurements after ATP-synthase inhibition with oligomycin showed that GW4064-treated cells have a lower capacity to metabolize glucose, which translates into lower ATP-dependent oxygen consumption. Altogether, these results show that FXR activation decreases the transcription of glycolytic enzymes not only in human hepatocytes [12] , but also in enteroendocrine L cells leading to a decrease in intracellular ATP levels and ATP-dependent GLP-1 secretion in response to glucose. An increasing body of evidence shows that BA pool size and composition control glucose homeostasis through BA receptors. Although their action through the transmembrane receptor TGR5 is likely to occur rapidly after food ingestion, activation of the nuclear receptor FXR induces a more delayed response thus leading to a shift between early postprandial positive effects of TGR5 activation and delayed effects through FXR activation. FXR activation in the intestine increases FGF15/19 secretion which, in addition to its role in the regulation of BA synthesis, reduces adiposity, increases brown adipose tissue energy expenditure and improves the metabolic rate in different obese murine models [37] , [38] . In contrast, recent studies in obese mice highlight that intestinal FXR antagonism results in improved energy homeostasis [15] , [16] , [39] . Indeed, recently identified as endogenous BA FXR antagonists in GF mice [17] , TβMCA and TαMCA inactivate intestinal FXR [15] , [39] and protect mice against diet-induced obesity and improve glucose metabolism [15] , [39] . Treatment of GLUTag cells with CDCA, a natural FXR agonist, decreased, whereas TβMCA increased proglucagon gene expression. In agreement with these findings, GF mice express higher intestinal levels of proglucagon than CONV-R mice [40] . In addition, we show here that the increase of intestinal proglucagon mRNA upon FXR deficiency requires the gut microbiota since FXR deficiency in GF mice does not further enhance proglucagon mRNA levels. Assessing the dialogue between bile acids, gut microbiota and FXR in L cells could be an interesting way to increase GLP-1 production. Whole-body and intestinal FXR-deficient mice are protected against obesity and have an improved glucose metabolism [14] , [15] . By using the GLP-1R antagonist Exendin-4(9-39), we demonstrate that the improved glucose metabolism in Fxr−/− mice fed a HFD implies the GLP-1 pathway. BASs are resins which complex BA, preventing ileal BA re-absorption and driving BA to the colon thus facilitating their elimination [41] , [42] . Initially used for their cholesterol-lowering effect, BAS treatment has been shown to lower blood glucose in T2D patients (for review, see ref. 43 ). Among the proposed mechanisms, FXR deactivation increases energy expenditure in obese mice [2] , [14] , [41] . Another mechanism may rely on the TGR5-mediated increase in GLP-1 production and secretion. In the colon, which contains the highest density of GLP-1 expressing cells, BAS-bound BA increase proglucagon mRNA levels and meal-induced GLP-1 secretion thus improving glucose metabolism in high-fat-fed mice [20] , [21] . In this study, we demonstrate a role also for FXR in the response to colesevelam resulting in an increase of proglucagon mRNA levels in ileum and colon translated to an improved response to oral glucose suggesting that compounds with TGR5 agonist–FXR antagonist activity may be most optimal to enhance incretin production. Taken together, our results demonstrate that FXR activation decreases glycolysis and ATP production, which, in turn, decreases proglucagon transcription and GLP-1 secretion in response to glucose. In pathophysiological conditions, the beneficial effect of FXR deficiency is, at least in part, related to this newly identified FXR/GLP-1 pathway. Our study further provides a novel molecular mechanism contributing to the beneficial effects of BAS on glucose control in T2DM through increased GLP-1 production upon FXR deactivation in intestinal L cells ( Fig. 9 ). Thus, inhibiting FXR in L cells through a change in BA pool composition or through combination TGR5-agonist and FXR-antagonist treatment could be a promising approach to treat T2DM. 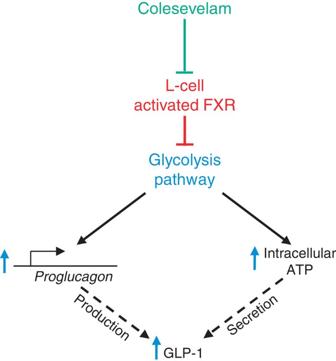Figure 9: Proposed mechanism by which L-cell FXR decreases GLP-1 production and secretion. Glucose induces proglucagon gene expression in L-cells via the glycolysis pathway and ChREBP, and subsequently promotes GLP-1 production. Moreover, glycolysis increases intracellular ATP concentrations and induces GLP-1 secretion. FXR activation, by inhibiting glucose metabolism, decreases both GLP-1 production and secretion. Colesevelam, by inhibiting FXR transcriptional activity in L-cells, promotes GLP-1 production and secretion. Figure 9: Proposed mechanism by which L-cell FXR decreases GLP-1 production and secretion. Glucose induces proglucagon gene expression in L-cells via the glycolysis pathway and ChREBP, and subsequently promotes GLP-1 production. Moreover, glycolysis increases intracellular ATP concentrations and induces GLP-1 secretion. FXR activation, by inhibiting glucose metabolism, decreases both GLP-1 production and secretion. Colesevelam, by inhibiting FXR transcriptional activity in L-cells, promotes GLP-1 production and secretion. Full size image Chemicals and reagents The DPP-4 inhibitors diprotin A, FFA-free bovine serum albumin (BSA), CDCA, TβMCA, exendin-4(9-39), phloretin, DMSO and CMC were purchased from Sigma-Aldrich (St Quentin-Fallavier, France). Sitagliptin was purchased from MSD. The synthetic FXR agonist GW4064 was purchased from Tocris (R&D Systems, Lille, France). For in vitro or ex vivo experiments, CDCA, TβMCA and GW4064 were dissolved in dimethylsulfoxide (DMSO) at 0.1% final. For in vivo experiments, GW4064 was dissolved in 1% carboxymethylcellulose (CMC) and Exendin-4(9-39) was dissolved in NaCl 0.9%. Chow and high fat diets were purchased from UAR (A04, Villemoison/Orge, France). Colesevelam–HCl was a kind gift of Daiichi Sankyo. Animal models and experimental protocols Eight-week-old C57Bl6/J male Fxr+/+ , Fxr−/− , ob/ob Fxr+/+ , ob/ob Fxr−/− littermates (INSERM U1011), 12-week-old C57Bl6/J male Tgr5−/− (CNRS/INSERM/ULP, Illkirch) and WT mice (Charles River Laboratories, Wilmington, MA), fed a chow diet, were housed in a temperature-controlled room (22 °C) on a 12-h light–dark cycle. GLU-VENUS, germ-free (GF) and conventionally raised (CONV-R) mice were housed as previously stated [17] , [40] . Wild-type (eight mice per group) and Tgr5−/− (five mice per group) mice were gavaged for 5 days with 1% CMC containing or not GW4064 (30 mpk). After randomization in four groups based on age and body weight, C57Bl6/J male mice deficient ( Fxr−/− ) or not ( Fxr+/+ ) for FXR were fed a standard chow diet (five to six mice per genotype) or a high-fat diet (12 mice per genotype). Age-matched C57Bl6/J male mice germ-free (GF) or conventional raised (CONV-R), on Fxr+/+ or Fxr−/− backgrounds (11–12 mice per group) were fed a standard chow diet (Labdiet). Eight-week-old C57Bl6/J male Fxr+/+ and Fxr−/− mice on a leptin-deficient ( ob/ob ) background (six to seven mice per group) were fed ad libitum during 3 weeks with a standard diet (UAR A04, Villemoison/Orge, France) supplemented or not with 2% of colesevelam–HCl. Eight-week-old Fxr+/+ and Fxr−/− mice (12 mice per genotype) received a HFD (D12492; Research Diets; 60% kcal fat) and controls received a chow diet for 6 weeks. Body weight was monitored weekly and glucose tolerance tests were measured as previously described [14] . Briefly, after 6 h fasting, mice were injected with NaCl 0.9% ( n =6 mice per group) containing or not Exendin-4(9-39) (0.5 mpk, n =6 mice per group) 45 min before intragastric glucose gavage (2 g kg −1 ). One week later, the same mice were subjected to intraperitoneal glucose injection (2 g kg −1 ). Glycaemia were measured at 0, 15, 30, 60, 90 and 120 min after either glucose gavage or intraperitoneal injection. For the in vivo GLP-1 experiments, mice were fasted 6 h, gavaged with sitagliptin (25 mpk) 45 min before a glucose bolus (2 g kg −1 ). Fifteen minutes after glucose gavage, blood (250 μl) was sampled by retro-orbital venipuncture under isoflurane anaesthesia and plasma GLP-1 was measured as described below. After 6 h fasting, mice were killed by cervical dislocation. Ileum (corresponding to the five terminal centimetres of the small intestine) and colon were washed once with phosphate-buffered saline (PBS), opened longitudinally on ice and the intestinal mucosa was scrapped and snap-frozen in liquid nitrogen. The experiment on GLU-VENUS mice was approved by local ethics committees and conformed to United Kingdom Home Office regulations, the experiment on Tgr5−/− mice were approved by the local animal experimentation committee of the Canton de Vaud (license no. 2614) and the experiment on GF/CONV-R mice was performed with protocols approved by the University of Gothenburg Animal Studies Committee. All the other experimental protocols were approved by the Lille Pasteur Institute Ethical committee and carried out in agreement with European Union (EEC no. 07430). Ex vivo studies GLP-1 secretion on murine intestinal biopsies . Murine ileal biopsies from WT mice treated for 5 days with CMC or GW4064 (30 mpk) were isolated as previously described [4] . Briefly, after 6 h fasting, mice were killed by cervical dislocation. The last 8 cm of the small intestine, corresponding to the ileum, was placed in cold Hank’s Balance Salt Solution (HBSS, Lonza) containing 2% horse serum (Life Technologies). Peyer’s patches were removed and the ileum was opened longitudinally and cut into 5-mm-long pieces. Pieces were washed 5 × in cold HBSS plus 2% horse serum and then incubated for 10 min at 4 °C in HBSS containing 2% horse serum and 1,4-dithiothreitol (DTT, 1 mmol l −1 ). After additional washing in cold HBSS plus 2% horse serum, ileum pieces were distributed in 48-well plates and stabilized for 3 h at 37 °C in Iscove’s Modified Dulbecco Medium (Life Technologies) containing 10% fetal calf serum (Life Technologies). After 30 min glucose deprivation in DMEM No Glc medium, a 1 h-GLP-1 secretion test in response to DMEM without glucose, to DMEM with glucose (5.5 mmol l −1 ) or in response to DMEM with glucose (5.6 mmol l −1 ) plus phloretin (0.5 mmol l −1 ) was performed at 37 °C in DMEM plus 1% DPP-4 inhibitor (Ile-Pro-Ile, Sigma-Aldrich). Finally, medium was removed, centrifuged for 5 min at 4 °C at 13,000 g and immediately frozen at −80 °C. GLP-1 content in culture medium was measured as described below. The remaining tissue was washed in cold PBS and frozen at −80 °C in NaOH 2 N. Protein content was assessed according to BCA’s method (Thermoscientific). Culture and immunostaining on human intestinal biopsies . Fresh human jejunum biopsies from normoglycemic subjects were obtained with informed consent as part of the A Biological Atlas of Severe Obesity (ABOS) study (ClinicalTrials.gov; NCT01129297). Mucosa were dissociated from musculosa and cut into small pieces of 1 cm 2 before treatment for 16 h with DMSO or GW4064 (5 μmol l −1 ) in RPMI medium+GlutaMAX-1 (catalogue (Cat.) No. 61870-010, Life Technologies) containing glucose (11 mmol l −1 ), sodium pyruvate (1 mmol l −1 ) and supplemented with 10% FBS (Life Technologies) and penicillin/streptomycin (10,000 U l −1 per 10 mg l −1 ) in a 37 °C, 5% CO 2 controlled atmosphere. RNA extraction and qPCR analysis were performed as described below. For immunohistochemical analysis, human jejunal biopsies were overnight (O/N) fixed with paraformaldehyde 4% (Sigma) before incubation with 20% sucrose during 20 h and further inclusion in Jung Tissue Freezing Medium (Jung) and storage at −80 °C before processing. Twelve-micrometre-thick slices were post-fixed in methanol/acetone 50/50 (v/v) for 10 min at −20 °C. After two washes in Tris/NaCl buffer (TRIZMA-Base (20 mmol l −1 , Sigma)/NaCl (150 mmol l −1 , VWR), pH 7.6), an antigen retrieval step was performed (520 W, 5 min; 160 W, 10 min) in citrate buffer (ThermoScientific). After permeabilization during 10 min (Tris/NaCl/0.1% TRITON X100), unspecific protein binding sites were masked by Dako Protein Block (DAKO) during 2 h at room temperature. Then, the samples were incubated O/N with mouse anti-human GLP-1 (SC-73508, Santa Cruz Biotechnology) and rabbit anti-human FXR (Ab28676, Abcam) antibodies (1/100) at 4 °C. The next day, immunoreactive cells were revealed after incubation with goat anti-mouse IgG Alexa 568 (for GLP-1) and goat anti-rabbit IgG Alexa 488 (for FXR; dilutions: 1/200, Molecular Probes) and photographies were taken with a confocal microscope (LSM 710 Zeiss). Image analysis was performed using the ImageJ software (version 1.46c; WS Rasband, National Institutes of Health, Bethesda, MD, USA, http://rsb.info.nih.gov/ij/ ). In vitro studies Cell culture and treatment . The mouse enteroendocrine L cell line GLUTag was kindly provided by D.J. Drucker (University of Toronto, Toronto, Canada) and grown in DMEM+GlutaMAX-1 medium (Cat. No. 21885-025, Invitrogen) containing glucose (5.6 mmol l −1 ), sodium pyruvate (1 mmol l −1 ) and supplemented with 10% FBS. For treatments, 42 h cultured cells were incubated for 24 h in DMEM+GlutaMAX-1 medium (Cat. No. 21885-025, Invitrogen) with glucose (5.6 mmol l −1 ), sodium pyruvate (1 mmol l −1 ) and supplemented with 0.2% BSA containing TβMCA (100 μmol l −1 ), CDCA (100 μmol l −1 ) or GW4064 (5 μmol l −1 ) during 24 h unless specified. In some experiments, cells were deprived of glucose by a 12 h incubation in glucose-free medium (DMEM GLUTamax, Cat. No. 11966-025), supplemented with 1% glutamine, sodium pyruvate (1 mmol l −1 ), 0.2% BSA and sodium lactate (10 mmol l −1 ) before FXR activation in either lactate (10 mmol l −1 )-, glucose (5.6 mmol l −1 )- or 2-deoxyglucose (5.6 mmol l −1 )-containing medium. Transient transfection assays . Cells were electroporated using the Neon Transfection System (Life Technologies) with small interference RNA against random (siCtrl), Fxr (si Fxr ) or Mlxipl (si Chrebp ) sequences (smart pool sequences obtained from Dharmacon (Thermoscientific, Illkirch, France); see Table 1 ). A total 140,000 electroporated cells cm −2 seeded into 24-well plates during 42 h were treated as described above. Table 1 Mouse small interfering RNA sequences used in siRNA experiments. Full size table GLP-1 secretion assays, ATP and mitotracker-FACS measurement . After treatment, GLUTag cells were starved for 30 min in glucose-free Krebs/phosphate buffer (NaCl (120 mmol l −1 ), KCl (5 mmol l −1 ), MgCl 2 (0.25 mmol l −1 ), CaCl 2 (0.5 mmol l −1 ) and NaHCO 3 (2.2 mmol l −1 ), pH 7.2) supplemented with diprotin A (100 μmol l −1 ) and 0.2% BSA. Cells were subsequently stimulated for 1 h with Krebs buffer with or without glucose (5.6 mmol l −1 ) or with a Krebs buffer enriched with KCl (30 mmol l −1 ). The cell supernatants were then transferred into ice-cold microtubes containing an equal volume of diprotin A (100 μmol l −1 ) in Krebs buffer and centrifuged at 1,500 g , 4 °C for 5 min. Cells were lysed in NaOH (0.8 mol l −1 ) under agitation and total protein content was determined using the BCA Protein Assay Kit (Pierce). Active 7-37 and 7-36 amide GLP-1 were measured with an enzyme-linked immunosorbent assay kit (EGLP-35K; Merck-Millipore) using Mithras Technology (Berthold) and normalized to the total quantity of cellular proteins. ATP measurement (Cell Titre Glow, Promega) on GLUTag cells in response to glucose (5.6 mmol l −1 ) was performed in the same condition as GLP-1 secretion assays according to the manufacturer’s protocol and luciferase activity was measured using Viktor apparatus (PerkinElmer). To estimate mitochondrial quantity, 24 h DMSO- and GW4064-treated GLUTag cells were washed with PBS, trypsinized and incubated at 37 °C for 20 min with 100 nmol l −1 MitoTracker Green FM (Molecular Probes). Samples were washed 3 × in PBS and subjected to flow cytometric analysis on a FACSCalibur apparatus (Becton Dickinson, San Jose, CA). Analysis of oxygen consumption and glycolytic rates . Measurements of OCR and ECAR in GLUTag cells were performed using the XF24 analyser (Seahorse Bioscience). A total 4 × 10 4 GLUTag cells per well were seeded in XF24 V7 microplates for 42 h before GW4064 treatment for 24 h. OCR and ECAR were measured in Seahorse assay buffer containing basic glucose-free DMEM medium (pH 7.4). The following compounds and concentrations were added successively: glucose (10 mmol l −1 ); oligomycin (1 μmol l −1 ); 2-deoxyglucose (100 mmol l −1 ); rotenone (1 μmol l −1 ) and antimycin A (1 μmol l −1 ). Co-immunoprecipitation and western blot analysis . GLUTag cells were glucose-deprived for 12 h and then treated 24 h with DMSO or with GW4064 (5 μmol l −1 ) in the presence of lactate (10 mmol l −1 ) or glucose (5.6 mmol l −1 ). After three washes in ice-cold PBS, cells were scrapped in ice-cold PBS containing protease inhibitors (1 × , Roche). Cells were centrifuged for 5 min at 3,500 g at 4 °C. One volume of the cell lysis buffer (KCl (10 mmol l −1 ), TRIS HCl pH 7.9 (10 mmol l −1 ), DTT (0.5 mmol l −1 ), MgCl 2 (1.5 mmol l −1 ), PIC 0.1%), corresponding to the cell volume was added and cells were incubated on ice during 15 min. Cells were then centrifuged for 1 min at 11,500 g at 4 °C. Supernatants were collected (that is, cytoplasmic fraction) and pellets were lysed in modified RIPA buffer (TRIS HCl pH 7.4 (50 mmol l −1 ), NaCl (150 mmol l −1 ), 0.25% DOC, 0.5% NP40, EDTA (1 mmol l −1 ), 0.1% PIC) 30 min on ice. After centrifugation (5 min at 13,000 g at 4 °C) supernatants corresponding to the nuclear fraction were collected. After a pre-clearing step in which protein fractions were incubated with protein A agarose beads (1 h 30 min at 4 °C), cells were centrifuged (5 min at 1,000 g at 4 °C) and 200 μg of protein were immunoprecipitated (O/N at 4 °C) with antibody against FXR (2 μg). Then immunocomplexes were captured with 100 μl protein A agarose beads 3 h at 4 °C, centrifuged 1 min at 1,000 g and washed three times with 800 μl of RIPA modified buffer. Beads were resuspended in 2 × migration buffer and heated for 3 min at 100 °C. Western blots were generated as previously described [29] and incubated with proglucagon (SC-80730, Santa Cruz), FXR (PP-9033A, R&D), ChREBP (Novus Biological, NB400-135) or β-actin (SC-1616, Santa Cruz) antibodies (diluted: 1/500). After 1 h incubation with horseradish peroxydase-conjugated secondary antibodies (1/3,000, Sigma), protein revelation was performed using the enhanced chemiluminescence FEMTO Plus reagents (ECL FEMTO, Thermofischer) by autoradiography (Camera Gbox, SynGene) and band intensity was measured (GeneTools software, SynGene). Microarray analysis . GLUTag cells were treated or not with GW4064 (5 μmol l −1 ) for 24 h and four RNA samples of each treatment condition were hybridized on mouse GEP 8 × 60 K arrays. Scanning clusters and data acquisition were carried out following the manufacturer’s instructions (Agilent, One-colour microarray Gene Expression Analysis). Data processing and analysis were performed using the Genespring Software. Biological Processes Analysis was performed using Gene Ontology Biological Processes on the Genomatix Software (Genomatix, Deutschland). Data are deposited at EBI under the E-MTAB-2199 number. RNA extraction and quantification by qPCR Total RNAs from FACS-isolated cells were isolated using a micro-scale RNA isolation kit (RNAeasy, Qiagen, Crawley, UK) and were reverse transcribed according to standard protocols using a Peltier Thermal Cycler-225 (MJ Research, Waltham, MA, USA). Quantitative PCR with reverse transcription was performed with 7900 HT Fast Real-Time PCR system (Applied Biosystems, Foster City, CA, USA). PCR reactions mix consisted of first-strand cDNA template, primers (TaqMan gene expression assays, Applied Biosystems) and PCR Master mix (Applied Biosystems). Fxr gene expression was compared with that of β-actin measured on the same sample, in parallel, on the same plate, giving a cycle threshold difference (ΔCT) for Fxr gene minus β-actin. Total RNAs from GLUTag cells, mouse and human epithelial cells were extracted using Extract-All Reagent (Eurobio, Courteboeuf, France) according to the manufacturer’s protocol. After DNAse treatment (Fermentas, St Rémy Les Chevreuse, France), total RNA (0.5–1 μg) was reverse transcribed using High-Capacity Multiscribe Reverse Transcriptase (Applied Biosystems, St Aubin, France) according to the manufacturer’s protocol. qPCR with reverse transcription was performed using the Master MIX SYBR Green Brillant Fast III (Agilent) on a MX4000 apparatus (Stratagene) using specific oligonucleotides (see Table 2 ). The results are presented using the ΔΔCt method normalized to a reference gene (Cyclophilin for in vitro and ex vivo experiments and TFIIB for in vivo experiments). Controls were set at 1 and all conditions were expressed comparatively to control. Table 2 qPCR primer sequences. Full size table Data analysis In vitro experiments were performed in triplicates and repeated at least three times. The in vitro and ex vivo data are presented as mean±s.d. The in vivo data are presented as mean±s.e.m. All statistical analyses were performed using two-tailed Student’s t -test or one-way analysis of variance followed by Tukey’s post hoc test or two-way analysis of variance followed by Bonferronni’s post hoc test and stated in the figure legends. P values ≤0.05 were considered as significant. How to cite this article: Trabelsi, M.S. et al. Farnesoid X receptor inhibits glucagon-like peptide-1 production by enteroendocrine L cells. Nat. Commun. 6:7629 doi: 10.1038/ncomms8629 (2015).